Enhanced electromechanical response of ferroelectrics due to charged domain walls While commonly used piezoelectric materials contain lead, non-hazardous, high-performance piezoelectrics are yet to be discovered. Charged domain walls in ferroelectrics are considered inactive with regards to the piezoelectric response and, therefore, are largely ignored in this search. Here we demonstrate a mechanism that leads to a strong enhancement of the dielectric and piezoelectric properties in ferroelectrics with increasing density of charged domain walls. We show that an incomplete compensation of bound polarization charge at these walls creates a stable built-in depolarizing field across each domain leading to increased electromechanical response. Our model clarifies a long-standing unexplained effect of domain wall density on macroscopic properties of domain-engineered ferroelectrics. We show that non-toxic ferroelectrics like BaTiO 3 with dense patterns of charged domain walls are expected to have strongly enhanced piezoelectric properties, thus suggesting a new route to high-performance, lead-free ferroelectrics. In the last two decades, sensors and actuators based on lead-containing ferroelectrics gained a dominant position in applications ranging from delicate positioning systems, ultrasonic medical diagnostic tools and microsurgery devices to robust fuel injectors. These lead-containing materials have to be replaced by environmentally benign alternatives [1] , [2] . So far, the search for lead-free ferroelectrics was mainly focused on the synthesis of new compositions exhibiting high-intrinsic piezoelectric properties [3] , [4] , [5] . The possibility to enhance piezoelectric properties of known lead-free ferroelectric crystals by so-called frustrated poling and domain engineering has also been explored [6] , [7] , [8] , [9] , [10] . In this approach, the poling electric field is applied along a nonpolar direction, which forms equal angles with at least two possible orientations of spontaneous polarization. During this poling, two or more ferroelectric states are equally preferred, creating an artificial domain structure with several coexisting domain states. Such a structure is macroscopically polar (has non-zero net polarization) and includes a certain volume fraction of domain walls. It has been found that, in the classical lead-free perovskite ferroelectric BaTiO 3 , a high density of domain walls with spacing in the micrometre range can result in up to a fourfold enhancement of functional properties [9] , while it was established that the enhancement is not associated with the domain wall motion. However, the body of available experimental data is insufficient to clearly relate the observed effects to features of the domain patterns in the samples. This experimental activity has drawn much attention by theorists [11] , [12] , [13] , [14] , [15] who were unable to explain the experimental observations unless unrealistic assumptions were taken. Thus, despite intriguing experimental findings, the future of fine-scale domain patterns as systems with enhanced electromechanical properties remains obscure. Here we demonstrate the existence of an enhancement mechanism of the dielectric and piezoelectric response in ferroelectrics with fine-scale charged domain-wall patterns. This mechanism provides a realistic interpretation of the experimental observations and outlines a new direction in the search for high electromechanical response in lead-free ferroelectrics. In the experimental reports on enhanced properties due to engineered domain structures, we recognized that head-to-head and tail-to-tail domain configurations [16] , [17] , [18] , [19] , such as those shown in Fig. 1 , must have been formed during the frustrated poling process of BaTiO 3 (refs 8 , 10 ). The reports [8] , [10] describe poling techniques leading to the controlled formation of domain structures with various domain-wall densities. Analysis of the domain walls and crystal orientations leads to indirect identification of 90°-charged domain walls [10] which occupy an unspecified fraction of crystal volume. However, the significance of this formation of charged domain walls passed entirely un-noticed. 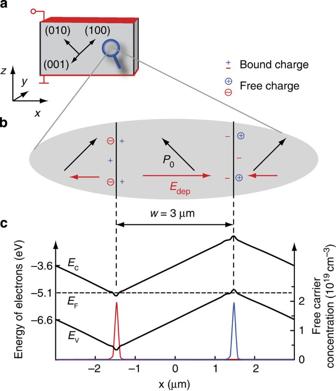Figure 1: Free carrier concentration and band bending at charged domain walls. (a) An electroded (110)cplate of tetragonal BaTiO3. (b) A periodic structure of charged 90° domain walls where bound polarization charge (+, −) induced by divergence of polarization,P0, is almost perfectly compensated by free charge (,) whereas the imperfection of compensation creates built-in depolarizing fieldEdep. (c) Phase-field simulation-calculated band bending induced byEdep. The bending causes the edges of the conductionECor valenceEVbands (solid black lines) to approach the Fermi levelEF(dashed black line) where high concentration of free electrons (red line) or holes (blue line) are generated and become available for compensation of the bound charge. The bandgap between the conduction and valence bands is assumed 3 eV. The competing band bending and charge compensation are in equilibrium when conduction and valence bands cross the Fermi level about ~0.22 eV at head-to-head and tail-to-tail domain walls, respectively. Figure 1: Free carrier concentration and band bending at charged domain walls. ( a ) An electroded (110) c plate of tetragonal BaTiO 3 . ( b ) A periodic structure of charged 90° domain walls where bound polarization charge (+, −) induced by divergence of polarization, P 0 , is almost perfectly compensated by free charge ( , ) whereas the imperfection of compensation creates built-in depolarizing field E dep . ( c ) Phase-field simulation-calculated band bending induced by E dep . The bending causes the edges of the conduction E C or valence E V bands (solid black lines) to approach the Fermi level E F (dashed black line) where high concentration of free electrons (red line) or holes (blue line) are generated and become available for compensation of the bound charge. The bandgap between the conduction and valence bands is assumed 3 eV. The competing band bending and charge compensation are in equilibrium when conduction and valence bands cross the Fermi level about ~0.22 eV at head-to-head and tail-to-tail domain walls, respectively. Full size image Here we report an analysis, based on Landau–Ginzburg–Devonshire theory and the theory of semiconductors, which establishes that the dielectric and piezoelectric response of such systems with charged domain walls increase strongly on the reduction of the domain period. This is expected to happen under two conditions: the ferroelectric phase transition in the material should be of first order and a strong dielectric anisotropy must exist, namely the dielectric constant in the direction perpendicular to the spontaneous polarization, a , should be much larger than that in the direction parallel to it, c . Both these conditions are met for BaTiO 3 (ref. 20 ) and KNbO 3 (ref. 21 ). Charged domain walls Charged domain walls contain a high density of bound charges, which must be strongly compensated by free carriers to prevent a huge depolarizing field that would prohibit formation of dense periodic domain structures. For realistic parameters of ferroelectric perovskites (unless these are heavily doped), such compensation cannot be provided with the typical carrier concentration in these materials [16] , [22] . Most of the screening charge originates from electron transfer across the forbidden energy gap, E g . This means that, at the head-to-head wall (positive bound charge), the bottom of the conduction band of the material should approach the Fermi level, providing electrons for the screening. Analogously, at the tail-to-tail wall (negative bound charge), the top of the valence band approaches the Fermi level, providing screening holes. This implies the existence of a potential difference of about E g / q ( q is the elementary charge) between such couple of walls. As a result, the domain between these walls is exposed to an electric field, E dep , which depends on the forbidden gap and the domain width, w , as expressed in equation (1), This field is a result of the incomplete compensation of bound polarization charge with free carriers at the domain walls. The imperfect compensation is a principal feature of the system because a perfect compensation would result in zero-band bending, and then the free carriers needed for compensation would not be available at all. Therefore, the system keeps an optimal trade-off between imperfect screening and a minimal necessary band bending. In the case of an electroded (110) c (the subscript c denotes the pseudocubic orientation) plate of tetragonal BaTiO 3 ( Fig. 1a ) containing a pattern of charged domain walls ( Fig. 1b ), E g =3 eV and with domain width w of several micrometres, the depolarizing field E dep can readily reach values of 10–20 kV cm −1 (equation (1)). It is this built-in field (growing with domain-wall density) that induces a polarization rotation leading to enhanced dielectric and piezoelectric response of each domain. Polarization rotation The mechanism of polarization rotation is qualitatively illustrated in Fig. 2 for the case of tetragonal BaTiO 3 . The contour plot of bulk free-energy density, Fig. 2a , shows two global minima corresponding to two different orientations of polarization in the tetragonal phase and one local minimum for the orthorhombic phase. The minimal energy path for polarization switching between the two tetragonal states inevitably follows a rotation-like path across the orthorhombic minimum. The key factor responsible for the enhanced properties is that polarization rotated by E dep approaches a point of instability between tetragonal and orthorhombic phases. At this point, a small excitation by an external electric field in the [110] c direction is able to induce a large change of polarization along the dash-dotted line in Fig. 2 . The essential characteristic of a material that allows the enhancement effect is illustrated in Fig. 2b . It shows a surface that encloses a region where values of polarization lead to energy lower than −2.18 MJ m −3 . Polarization is stable in the tetragonal minima (white circles), but follows a minimal energy path during switching between the tetragonal states. The important feature is the non-zero change of the P 3 -component during switching. The energy profile corresponds to BaTiO 3 , but a qualitatively equivalent situation is available, for example, in a (111) c plate of KNbO 3 . 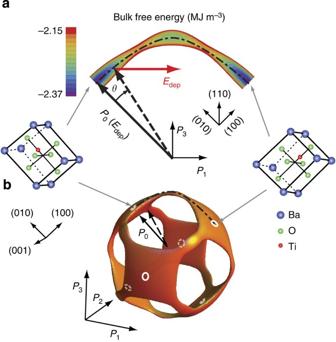Figure 2: Enhancement of the dielectric response by polarization rotation. The path for the rotation of the polarization vectorP0, which is induced by electric fieldEdep, is given by the profile of the bulk free energy (a). The dash-dotted line illustrates a path with minimal energy barrier for switching between domain states of the tetragonal phase (end points of the dash-dotted line). The key feature of the illustrated mechanism is theEdep-induced polarization rotation by an angleθthat is accompanied by a change ofP3-component of the polarization, approaching the point of thermodynamic instability. The three-dimensional contour plot (b) shows the surface of a region where the values of spontaneous polarization give energy lower than −2.18 MJ m−3. The enhancement effect is available when the minimal energy paths between the tetragonal minima (white circles) are curved into theP3direction. Figure 2: Enhancement of the dielectric response by polarization rotation. The path for the rotation of the polarization vector P 0 , which is induced by electric field E dep , is given by the profile of the bulk free energy ( a ). The dash-dotted line illustrates a path with minimal energy barrier for switching between domain states of the tetragonal phase (end points of the dash-dotted line). The key feature of the illustrated mechanism is the E dep -induced polarization rotation by an angle θ that is accompanied by a change of P 3 -component of the polarization, approaching the point of thermodynamic instability. The three-dimensional contour plot ( b ) shows the surface of a region where the values of spontaneous polarization give energy lower than −2.18 MJ m −3 . The enhancement effect is available when the minimal energy paths between the tetragonal minima (white circles) are curved into the P 3 direction. Full size image In view of the strong dielectric anisotropy of BaTiO 3 (experimentally at room temperature a / c 30) (ref. 20 ), it is the value of a that controls the total dielectric response of the system. For this reason, we discuss the impact of the built-in field E dep on this quantity alone. Let us consider the case where the application of the field leads to small changes of the ferroelectric polarization. In this approximation, the relative reduction of the absolute value of the polarization can be evaluated as is ( P 0 is the spontaneous polarization) with the transverse component being γδP 0 where γ = a / c is the dielectric anisotropy factor. Using the polarization equation of state in the X–Z plane, one can readily describe an impact of the built-in field on a in terms of the following relation between the modified value of the transverse component of the dielectric constant a and δ : Here factors A and B can be readily expressed in terms of the coefficient of the Landau expansion [23] : for BaTiO 3 at room temperature A ≈0.3 and B ≈0.6. The sign of the coefficient B has an essential role in the enhancement mechanism and it can only be positive in materials that exhibit a first-order phase transition. The A -containing term in equation (2) describes the elongation and contraction of polarization, whereas the B -containing term controls the effect of polarization rotation. In the linear approximation, the rotation angle θ can be expressed in terms of relative change of the polarization δ : θ = γδ . Keeping this in mind, one sees that the positive sign of B implies that the polarization rotation leads to a permittivity enhancement. Conversely, if the ferroelectric transition in the material were of the second order, B would be negative and the polarization rotation would not lead to enhancement of permittivity. With a large value of γ , one concludes from the equation (2) that polarization rotation is the leading effect. The angle corresponding to substantial enhancement of a can be evaluated from the condition Bγθ 2 1, yielding | θ | 13° for BaTiO 3 . Such a level of polarization rotation can be reached under realistic values of the built-in field. This is clear from Fig. 3a , which shows the calculated dependence of θ on E dep . Thus for the domain pattern addressed, the electric field arising from incomplete compensation of the bound charge on head-to-head and tail-to-tail walls is strong enough to dramatically enhance the dielectric response of the system. Similar effects of enhancement of the dielectric and piezoelectric properties can be expected also in KNbO 3 and in ferroelectrics at their morphotropic boundary. 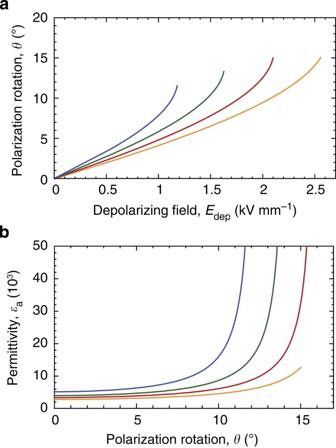Figure 3: Depolarizing field-induced polarization rotation and impact on permittivity. The angleθgrowing withEdep(a) which results in an increase of the transverse dielectric responsea(b). Displayed curves correspond to temperatures 278 K (blue), 288 K (green), 298 K (red), and 308 K (orange). Figure 3: Depolarizing field-induced polarization rotation and impact on permittivity. The angle θ growing with E dep ( a ) which results in an increase of the transverse dielectric response a ( b ). Displayed curves correspond to temperatures 278 K (blue), 288 K (green), 298 K (red), and 308 K (orange). Full size image The semi-quantitative arguments following from equation (2) are supported by more detailed Landau-theory calculations (see Methods ) that show the unlimited growth of the transverse component of the dielectric constant when approaching a critical angle as shown in Fig. 3b . Properties of ferroelectrics with charged domain walls We verified the enhancement mechanism described above by means of phase-field simulations of a poly-domain system, where the ferroelectric was treated as a wide-bandgap semiconductor in the effective mass approximation (see Methods ). First, stability of 90°-charged domain walls was confirmed. Then, we have calculated piezoelectric, d 33 and d 31 , and dielectric 33 coefficients as functions of domain-wall spacing w , which are experimentally measurable parameters of the system. The phase field results (circles and squares in Fig. 4a–c ) include contributions of domain response and intrinsic response of domain walls. To identify the magnitudes of these contributions, we performed the Landau-theory calculations for a single domain that is artificially exposed to depolarizing electric field applied along x axis ( Fig. 1b ). The magnitude of this electric field was obtained from phase-field simulation as approximately E dep =Δ V eff / w where Δ V eff =3.5 V is an 'effective' potential difference between domain walls. This potential difference is larger than E g /q = 3 V due to the shape of the band bending ( Fig. 1c ). However, as seen in Fig. 4a–c , the intrinsic domain wall contribution, which is the difference between single-domain and poly-domain response, is negligible. This conclusion is surprising with respect to the huge domain-wall thickness ( Fig. 4d ), but it agrees with studies done in the past [11] , [12] , [13] , where intrinsic domain-wall response failed to explain the experimental observations [7] , [8] , [9] , [10] . The large thickness of charged domain walls, DW >100 nm, compared with neutral ones, DW ~1 nm, is qualitatively consistent with a recently published theory [16] that explains the widening mechanism of charged domain walls in detail. Our calculations also show temperature T and E g dependence of the smallest theoretically possible domain-size w lim ( Fig. 4e ). 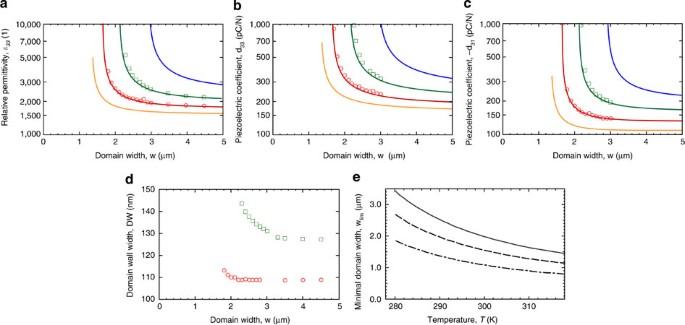Figure 4: Enhancement of macroscopic properties with decreasing domain size. Relative permittivity33(a), and piezoelectric coefficientsd33(b), andd31(c), are plotted as a function of domain widthw. The solid lines represent the inner response of a domain that is exposed to built-in depolarizing field owing to imperfectly compensated charged domain walls. Displayed curves correspond to temperatures 278 K (blue lines), 288 K (green lines), 298 K (red lines), and 308 K (orange lines). Red circles and green squares represent phase-field simulation results that include intrinsic contributions of charged domain walls at temperatures 288 K (green squares) and 298 K (red circles). Domain-wall widthDWagainst domain widthw(d), shows small domain-wall broadening when critical domain width is approached. (e) The critical (minimal) domain widthwlimagainst temperatureTis shown for bandgaps 2 eV (dash-dotted), 3 eV (dashed), and 4 eV (solid). Figure 4: Enhancement of macroscopic properties with decreasing domain size. Relative permittivity 33 ( a ), and piezoelectric coefficients d 33 ( b ), and d 31 ( c ), are plotted as a function of domain width w . The solid lines represent the inner response of a domain that is exposed to built-in depolarizing field owing to imperfectly compensated charged domain walls. Displayed curves correspond to temperatures 278 K (blue lines), 288 K (green lines), 298 K (red lines), and 308 K (orange lines). Red circles and green squares represent phase-field simulation results that include intrinsic contributions of charged domain walls at temperatures 288 K (green squares) and 298 K (red circles). Domain-wall width DW against domain width w ( d ), shows small domain-wall broadening when critical domain width is approached. ( e ) The critical (minimal) domain width w lim against temperature T is shown for bandgaps 2 eV (dash-dotted), 3 eV (dashed), and 4 eV (solid). Full size image The phase-field calculated band-bending profile and free-charge concentrations are shown in Fig. 1c , where the difference between the edge of the conduction (or valence) band and the Fermi level in the wall centre, Δ E , can be evaluated for the condition that the charge density of the free carriers at this point, ( m eff and ħ are the effective mass of electrones/holes, and the reduced Planck constant, respectively) is about the mean bound charge density in the walls, √2 P 0 / w . Such estimates, with m eff =0.12 m e ( m e is the free electron mass), w =100 nm and P 0 =0.26 C m −2 yield Δ E =0.24 eV in reasonable agreement with the results of phase-field simulation where Δ E ≈0.22 eV. The large concentration of free carriers at charged domain walls ( Fig. 1c ) may raise the question as to whether the expected high domain-wall conductivity cannot short-circuit the electrodes and hence make the enhancement phenomena practically unavailable. To answer this question, we simulated a finite–6 μm thick–electroded sample. One can see, in a colour-scale map in Fig. 5 , that the free-carrier concentration dramatically drops in the vicinity of the electrodes. This results in the formation of ~300 nm or ~1 μm gaps between electrodes and regions with higher free-charge concentration. These gaps are formed because of the flat profile of the electric potential (constant potential) at the electrodes that prohibits band-bending and, hence, a high concentration of free-carriers in the vicinity of the electrodes. The results in Fig. 5 correspond to the situation where the work functions of the electrode and ferroelectric are identical, but, in general, the size of the gaps is dependent on the difference between the work functions. 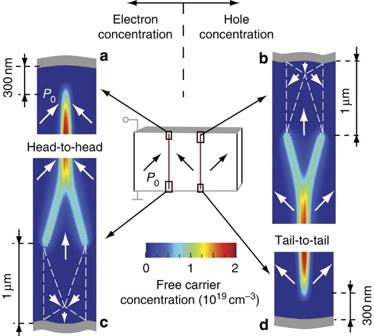Figure 5: Charged domain walls in the vicinity of electrodes. Colour-scale graphs show the distribution of free-carrier concentration in a ferroelectric with charged domain walls. The concentration is maximal in the centres of charged domain walls, but it dramatically drops in the vicinity of the electrodes. This results in a formation of ~300 nm (a,d), and ~1 μm (b,c), gaps between the electrodes and regions with higher free-charge concentration. These gaps are formed due to the flat profile of the electric potential (constant potential) at the electrodes that prohibits band-bending and, hence, a high concentration of free-carriers in the vicinity of the electrodes. The results correspond to the situation where the work functions of the electrode and ferroelectric are identical, but, in general, the size of the gaps is dependent on the difference between the work functions. Figure 5: Charged domain walls in the vicinity of electrodes. Colour-scale graphs show the distribution of free-carrier concentration in a ferroelectric with charged domain walls. The concentration is maximal in the centres of charged domain walls, but it dramatically drops in the vicinity of the electrodes. This results in a formation of ~300 nm ( a , d ), and ~1 μm ( b , c ), gaps between the electrodes and regions with higher free-charge concentration. These gaps are formed due to the flat profile of the electric potential (constant potential) at the electrodes that prohibits band-bending and, hence, a high concentration of free-carriers in the vicinity of the electrodes. The results correspond to the situation where the work functions of the electrode and ferroelectric are identical, but, in general, the size of the gaps is dependent on the difference between the work functions. Full size image Our analysis shows that the built-in electric field, created in periodic domain patterns with charged domain walls, grows significantly with increasing domain-wall density. Once the domain period is in the range of several micrometres, the built-in field can lead to an appreciable enhancement of the dielectric and piezoelectric response of the polydomain system. We identify the features that control this phenomenon, namely a very high dielectric anisotropy factor γ = a / c and a first-order ferroelectric phase transition. The presented results are qualitatively in good agreement with experimental observations of domain-wall density effects on macroscopic properties of [111] c -poled BaTiO 3 crystals [7] , [8] , [9] , [10] ( Fig. 6 ). In these experiments, the piezoelectric and dielectric constants were subject to a fourfold enhancement when domain size reached three-to-five microns. We suggest the presented mechanism as a new degree of freedom in the search for ferroelectrics with high piezoelectric response that is particularly attractive in light of the need for lead-free piezoelectrics. 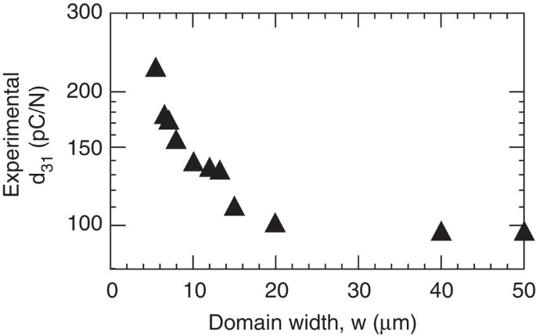Figure 6: Experimental data for the effect of domain density on macroscopic piezoelectric response. Experimental dependence of piezoelectric coefficientd31on domain sizewin poled (111)cplate of single crystal BaTiO3. Data are combined from refs9,10. Figure 6: Experimental data for the effect of domain density on macroscopic piezoelectric response. Experimental dependence of piezoelectric coefficient d 31 on domain size w in poled (111) c plate of single crystal BaTiO 3 . Data are combined from refs 9 , 10 . Full size image The phase-field model The presented results were obtained primarily by means of phase-field simulation that incorporates coupling between ferroelectric and wide-bandgap semiconductor properties. Our simulation includes elastic interactions that results in stable 90°-charged domain walls. Model equations are obtained by Lagrange principle from Helmholtz free-energy density [24] : where P i is the polarization, P i,j its derivatives (the subscript ',j' represents the operator of spatial derivatives ∂ / ∂x j ), D i the electric displacement and e ij =1/2( u i,j + u j,i ) is the elastic strain where u i is a displacement vector. The bulk free-energy density is expressed for a zero strain as a six-order polynomial expansion [13] , where α i , α ij (e) , α ijk are parameters fitted to the single-crystal properties ( Table 1 ). The remaining contributions represent bilinear forms of densities of elastic energy f ela [{ e ij }]=1/2c ijkl e ij e kl , where c ijkl is the elastic stiffness, electrostriction energy f es [{ P i , e ij }]=− q ijkl e ij P k P l , where q ijkl are the electrostriction coefficients, gradient energy f wall [{ P i,j }]=1/2 G ijkl P i,j P k,l , where G ijkl are the gradient energy coefficients, and electrostatic energy f ele [{ P i , D i }]=1/(2 0 B )( D i − P i ) 2 , where 0 and B are permittivity of vacuum and relative background permittivity, respectively. The zero-strain coefficients α ij (e) can be expressed in terms of usually introduced stress-free coefficients α ij as follows: Table 1 Values of material coefficients for BaTiO 3 used in the simulations. Full size table By using the Legendre transformation to electric enthalpy where E i = - , i is the electric field and the electric potential, and using Lagrange principle, we can uniformly express the set of field equations that govern the kinetics of ferroelectrics: Equation (5) defines the mechanical equilibrium while inertia is neglected. Equation (6) represents Gauss's law of a dielectric including a non-zero concentration of free electrons n and holes p . Equation (7) is the time-dependent Landau–Ginzburg–Devonshire equation [25] which governs the spatiotemporal evolution of spontaneous polarization with kinetics given by coefficient Γ. Coupling between the ferroelectric/ferroelastic system with its semiconductor properties is introduced by considering a non-zero density of free carriers (electron-hole) in the electrostatic equation (6). The semiconductor properties were introduced under the assumption of zero concentration of dopants, which was shown to be an acceptable approximation to a small concentration of defects and dopants [17] . The distribution of free carriers is governed by continuity equations: where electron and hole currents J i ( n ) and J i ( p ) , respectively, are governed by drift and diffusion as follows: . Here μ n and μ p are electron and hole mobilities, respectively. Because we analyse only the stationary solution in thermal equilibrium, we can introduce computationally convenient form of recombination rates R n and R p as follows: R n =−( n − n 0 )/ τ and R p =−( p − p 0 )/ τ , where τ is life-time constant and n 0 and p 0 are electron and hole concentrations in thermal equilibrium: Here F 1/2 is the Fermi-Dirac integral. Density of states is given by effective mass approximation: where effective mass m eff = cm e is assumed equal for electrons and holes. As the effective mass of free carriers in BaTiO 3 varies in literature, we tested the model with a wide range of effective mass constants, c 0.05, 50 , showing an insignificant impact on the enhancement phenomena. However, the constant c controls the screening regime (classical/degenerate) and width of the domain walls. Results presented in the graphs correspond to c =0.117, that is, N =10 24 m −3 used by Xiao et al . [26] The ferroelectric-semiconductor model was designed as a subdomain of size 2 w ×0.25(μm) 2 with applied periodic boundary conditions joining the solution of all solved variables between opposite parallel boundaries. The numerical solution of equations (5), (6), (7), (8) and (9) on the defined subdomain was performed by a finite element method with linear triangular elements of size 4 nm in the vicinity of domain walls and 40 nm inside domains. The simulation starts from initial conditions that are defined as zero for all variables except polarization which is , for P 0 =0.262 C m −2 , in regions separated by 70 nm gap, where P =(0,0). The simulation reaches thermal equilibrium in <5 ns and gives solutions for the spatial distribution of polarization P i , mechanical displacement u i , electric potential ϕ , and concentrations of electrons n and holes p . We used these to calculate the band-bending and charge concentrations in Fig. 1c and domain-wall width and critical domain size in Fig. 4d,e . Then the domain structure is exposed to (i) small compressive stress, 100 kPa, and (ii) small electric field, 4 V mm −1 , when the average change of electric displacement is integrated and (i) the direct piezoelectric and (ii) dielectric coefficients are calculated ( Fig. 4a–c ). This calculation also shows almost zero domain-wall widening when small electric field or stress are applied. The single-domain Landau-theory approximation The phase-field results are accompanied by Landau-theory calculations of a single domain, which is subjected to an artificially introduced depolarizing field obtained from the phase-field model. This approach calculates macroscopic properties of domains by minimization of Gibbs free energy. It allows domain wall and domain contributions to be distinguished. The Gibbs free energy of homogeneous stress-free sample is defined as Here the non-indexed symbols P , E represent vectors. The bulk free-energy density f bulk is defined as f bulk = f bulk (e) + f ela + f es for stress-free homogenous sample, that is, at e ij = Q ijkl P k P l . Here Q ijkl are the coefficients of the direct electrostriction effect. The calculation searches for the minimum of G ( P , E ) for non-zero electric field E that gives polarization as follows: Using P ( E ) and strain induced by electrostriction effect e ij ( E )= Q ijkl P k ( E ) P l ( E ), we calculate effective piezoelectric coefficients: where the starred symbols are expressed in the coordinate system of a (110) c crystal. The presented results correspond to phenomenological parameters as introduced in Table 1 . How to cite this article: Sluka, T et al . Enhanced electromechanical response of ferroelectrics due to charged domain walls. Nat. Commun. 3:748 doi: 10.1038/ncomms1751 (2012).